Defined TLR3-specific adjuvant that induces NK and CTL activation without significant cytokine productionin vivo Ligand stimulation of the Toll-like receptors (TLRs) triggers innate immune response, cytokine production and cellular immune activation in dendritic cells. However, most TLR ligands are microbial constituents, which cause inflammation and toxicity. Toxic response could be reduced for secure immunotherapy through the use of chemically synthesized ligands with defined functions. Here we create an RNA ligand for TLR3 with no ability to activate the RIG-I/MDA5 pathway. This TLR3 ligand is a chimeric molecule consisting of phosphorothioate ODN-guided dsRNA (sODN-dsRNA), which elicits far less cytokine production than poly(I:C) in vitro and in vivo . The activation of TLR3/TICAM-1 pathway by sODN-dsRNA effectively induces natural killer and cytotoxic T cells in tumour-loaded mice, thereby establishing antitumour immunity. Systemic cytokinemia does not occur following subcutaneous or even intraperitoneal administration of sODN-dsRNA, indicating that TICAM-1 signalling with minute local cytokines sufficiently activate dendritic cells to prime tumoricidal effectors in vivo . Double-stranded (ds) RNA is often a signature of viral infection, which induces production of type I interferon (IFN) and inflammatory cytokines [1] , [2] . Its putative analogue polyinosinic:polycytidylic acid (poly(I:C)) exhibits both strong antiviral and anticancer potential [3] , [4] . Poly(I:C) has been considered a promising adjuvant for cancer immunotherapy for several decades [4] , [5] , [6] . In mouse models, growth retardation of syngenic implant tumours is observed following administration of poly(I:C) [7] , [8] , which is due to dendritic cell (DC)-derived natural killer (NK) and cytotoxic T-cell (CTL) activity [9] , [10] . Nevertheless, it has not been successfully used therapeutically in patients with cancer [5] , [6] . The amount of poly(I:C) required for an adequate therapeutic response causes side effects, including arthlargia, fever, erythema and sometimes life-threatening endotoxin-like shock [5] , [6] , which have prevented application of this dsRNA analogue from the clinical use. These side effects may be related to cytokine storm induced by dsRNA, although the situation is somewhat alleviated when minimal poly(I:C)-LC (poly- L -lysine and methylcellulose) is used instead of effector-inducible doses of mere poly(I:C) alone [5] , [6] , [11] . According to recent understanding on pattern recognition of innate immunity, poly(I:C) is a ligand for multiple pattern recognition receptors (PRRs), including protein kinase R, retinoic acid-inducible gene-I (RIG-I), melanoma differentiation-associated gene 5 (MDA5) and Toll-like receptor (TLR) 3 (refs 1 , 4 , 12 ). Virus replication usually produces dsRNA within the cytoplasm of infected cells and stimulates the cytoplasmic RNA sensors [12] , [13] . In contrast, TLR3 is activated when dsRNA liberated from virus-infected cells is internalized into the endosome of non-infected phagocytes [4] , [14] , such as DCs and macrophages. Type I IFN and DC-mediated immune responses are evoked to suppress virus replication. Physiologically, these responses occur in a complex manner, therefore, what happens in vivo when only a single receptor is stimulated remains to be elucidated, whereas what happens in vivo when a single gene is disrupted has been reported in knockout (KO) mouse studies [1] . It is therefore crucial in drug design to create PRR ligands specific for each PRR for the development of immune adjuvant. Regression of tumour with a lesser major histocompatibility complex expression [15] is caused by reciprocal activation of NK cells by poly(I:C)-stimulated DC [9] , [16] . However, in antitumour immunity, constitutive proliferation of antitumour CTL is important and antigen (Ag)-presenting DC must capture not only innate patterns but also tumour-associated Ag (TAA) for their cross-priming [10] , [17] . CD8α + DC in mouse lymphoid tissue [10] , [18] , [19] and CD103 + and CD141 + DCs in humans [18] , [19] , [20] are representative subsets that express TLR3 and induce efficient Ag cross-presentation in response to dsRNA enabling presentation of Ags to CD8 + T cells on their major histocompatibility complex class I proteins. In contrast, interleukin (IL)-12, IL-6, tumour necrosis factor (TNF)-α and IFN-α/β are the main mediators released in the serum secondary to exogenously administered poly(I:C) [4] , [20] , [21] . Studies in KO mice suggested that TLR3 has a pivotal role in inducing cross-presentation [10] , [17] , but its role is marginal in systemic cytokine/IFN production in vivo [21] . Most cytokines (except IL-12 p40) and type I IFN detected in serum are attributable to poly(I:C)’s stimulation of RIG-I and/or MDA5, that is, the mitochondrial antiviral-signalling protein (MAVS) pathway [12] , [21] . CTL/NK cell activation and robust cytokine production can be assigned, although partly overlapping, to the TLR3/Toll-IL-1 receptor domain-containing adaptor molecule (TICAM)-1 or MAVS pathway, respectively. Here we generated synthetic dsRNA derivatives expected to specifically act on TLR3, but not on RIG-I/MDA5. These ligands exhibited strong activity in inducing antitumour CTL and NK cells and caused marked regression of tumours without off-target effects including significant increases of serum cytokine/IFN levels in mouse models. Design of novel TLR3 agonist What we experienced in developing an RNA adjuvant was that: very little in vitro transcribed dsRNAs entered the human cells [22] , whereas poly(I:C) as well as CpG or control GpC phosphorothioate oligodeoxynucleotides (sODNs) reached the endosome in human myeloid DCs and epithelial cells. Poly(I:C) and sODNs appeared to share the uptake receptor [23] . To deliver dsRNA to endosome TLR3, we have connected sODN to 5′ sense RNA and annealed it with antisense RNA ( Fig. 1a ) to guide dsRNA internalization into TLR3-positive endosomes. The RNA source was chosen from a vaccine strain of measles virus (MV), as children around the world undergo MV vaccination without severe adverse events. Because >40 bp dsRNA may be the minimal length for activation of TLR3 (ref. 24 ), we selected the region of defective interference RNA in the vaccine MV that causes no RNA interference [25] . 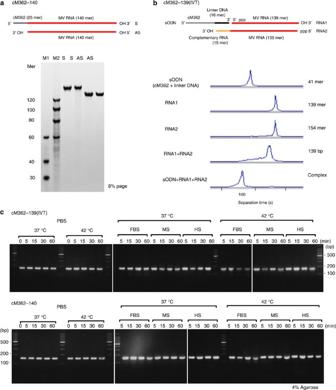Figure 1: Preparation of cM362-139 and cM362-140. (a) Schematic diagram of cM362-140. cM362-140 consists of chemically synthesized two nucleotide strands. The sense strand (S) is a 140 mer RNA capped with cM362 (25 mer) at 5′ site. The antisense strand (AS) is the complementary 140 mer RNA. Five pmol of S and AS RNAs were analysed on 8% PAGE containing 7M urea. M1 and M2, RNA size markers. (b) Schematic diagram of cM362-139(IVT) and its electropherograms. cM362-139(IVT) consists of three nucleotide strands, sODN (cM362+linker DNA; 41 mer),in vitrotranscribed sense RNA strand (RNA1; 139 mer) and antisense RNA strand (RNA2; 154 mer). All sequences of DNA and RNAs are described inSupplementary Tables. sODN, RNA1, RNA2, dsRNA (RNA1+RNA2) and complex cM362-139 (sODN+RNA1+RNA2) were analysed using multi-channel microchip electrophoresis. (c) Stability of cM362-139(IVT) and cM362-140. cM362-139(IVT) and cM362-140 were incubated in PBS with or without 10% heat-inactivated FBS, mouse serum (MS) or human serum (HS) at 37 °C or 42 °C for indicated time points. Aliquots containing 0.1 μg of treated cM362-dsRNAs were loaded onto a 4% agarose gel. Figure 1: Preparation of cM362-139 and cM362-140. ( a ) Schematic diagram of cM362-140. cM362-140 consists of chemically synthesized two nucleotide strands. The sense strand (S) is a 140 mer RNA capped with cM362 (25 mer) at 5′ site. The antisense strand (AS) is the complementary 140 mer RNA. Five pmol of S and AS RNAs were analysed on 8% PAGE containing 7M urea. M1 and M2, RNA size markers. ( b ) Schematic diagram of cM362-139(IVT) and its electropherograms. cM362-139(IVT) consists of three nucleotide strands, sODN (cM362+linker DNA; 41 mer), in vitro transcribed sense RNA strand (RNA1; 139 mer) and antisense RNA strand (RNA2; 154 mer). All sequences of DNA and RNAs are described in Supplementary Tables . sODN, RNA1, RNA2, dsRNA (RNA1+RNA2) and complex cM362-139 (sODN+RNA1+RNA2) were analysed using multi-channel microchip electrophoresis. ( c ) Stability of cM362-139(IVT) and cM362-140. cM362-139(IVT) and cM362-140 were incubated in PBS with or without 10% heat-inactivated FBS, mouse serum (MS) or human serum (HS) at 37 °C or 42 °C for indicated time points. Aliquots containing 0.1 μg of treated cM362-dsRNAs were loaded onto a 4% agarose gel. Full size image Because direct chemical synthesis of long sequences of RNA was unfeasible in our laboratory until recently, we first made the RNA duplex structures by in vitro transcription and annealing. sODN was connected via a linker DNA to dsRNA, so the three-chain structures were first designed ( Fig. 1b ) to carry forward by many trial-and-error tests for a specific TLR3 agonist. A GpC-type sODN cap cM362 ( Fig. 1a,b ) facilitates targeting to TLR3-positive endosomes, does not activate TLR9 and blocks dsRNA-mediated RIG-I/MDA5 activation; therefore it meets our criteria for a single PRR agonist. Testing function of in vitro transcribed sODN-dsRNAs Various kinds of sODN-dsRNA hybrid molecules were prepared by in vitro transcription and annealing ( Supplementary Fig. 1a , Supplementary Tables 1 and 2 ). In preliminary experiments to screen for a preferential sODN-dsRNA, we tested reporter gene (Luc125 for IFN-β promoter) activation in HEK293 cells expressing human TLR3. sODN-dsRNAs with dsRNA of >99 bp in length induced TLR3-dependent IFN-β-promoter activation similar to that induced by poly(I:C) in the presence or absence of fetal calf serum (FCS), whereas sODN-dsRNAs with dsRNA of <79 bp induced hardly any activation of TLR3 ( Supplementary Fig. 1b,c ). Notably, none of the sODN-dsRNAs examined were able to activate cytoplasmic RNA sensors when transfected into HEK293 cells ( Supplementary Fig. 2 ). We examined whether GpC motif or the length of sODN influenced the uptake of sODN-dsRNA. TLR3-mediated IFN-β promoter activation by sODN-dsRNA was independent of the presence of a GpC motif of sODN but dependent on the length; almost >20-mer of sODN is required for full activation of endosomal TLR3 ( Supplementary Fig. 3 ). 139 bp dsRNA and control B-type (c2006) or C-type (cM362) sODN were good candidates for activation of endosomal TLR3 with no TLR9 activation. We next examined the internalization of Cy3-labelled cM362-dsRNA (cM362-79, cM362-99 and cM362-139) in HeLa cells. cM362-dsRNAs were all similarly bound to the cell surface at 4 °C, but dsRNA73 and dsRNA139 without cM362 could not bind ( Supplementary Fig. 4 ). When cells were incubated at 37 °C, cM362-99 and cM362-139 both entered the cells more quickly than cM362 and cM362-79, localized in the early endosome after 15 min incubation and were retained for up to 120 min, whereas cM362 and cM362-79 co-localized with EEA1 at a later time point (30 min) and quickly moved to the lysosomes. Localization of cM362-139 in the lysosomes was observed after 60 min incubation, which was relatively slow compared with cM362-99 ( Supplementary Fig. 4 ). These results suggested that the length of dsRNA together with the presence of cM362 influences the internalization speed and retention time in the TLR3-situated early endosome. The abilities of cM362-dsRNAs to induce cytokine production were then examined using splenic DCs from wild-type and TLR3-deficient mice. cM362-79 and -139 induced a slight increase in TNF-α and IL-6 production by splenic CD11c + DCs in a TLR3-dependent manner ( Supplementary Fig. 5a ). Again, cM362-dsRNAs did not activate cytoplasmic RNA sensors in mouse splenic CD11c + DCs ( Supplementary Fig. 5b ). Thus, the chimeric compound cM362-139 appears to possess novel features that enable it to be quickly delivered to TLR3-positive endosomes, retained for a long period in the endosomes, and activate TLR3 but not RIG-like receptor (RLR). As a TLR3-specific agonist with high activity, we selected cM362-139 for further in vivo studies with tumour-loaded mice. Chemical synthesis of cM362-140 As chemical synthesis of sODN-dsRNA is indispensable for complying with good manufacturing practice (GMP) criteria, we started trials for chemical synthesis of cM362-140 ( Fig. 1a ), and its activity was analysed in comparison with in vitro transcribed cM362-139 ( Fig. 1a,b ). A synthesized 165 mer sense cM362-RNA hybrid and a 140mer antisense RNA, both of which consisted of single bands on 8% polyacrylamide gel electrophoresis (PAGE) and high-performance liquid chromatography/mass spectrometry analysis were annealed to make cM362-140 ( Fig. 1a , lower panel). First, the degradability of cM362-139(IVT) and chemically synthesized cM362-140 were tested under different conditions. Both compounds were stable during incubation in PBS with or without 10% FBS, mouse serum or human serum at 37 °C for 60 min. cM362-139(IVT) was slightly degraded in PBS containing FBS or mouse serum but not human serum during incubation at 42 °C ( Fig. 1c ). Notably, cM362-139(IVT) was susceptible to degradation by nucleases during incubation in RNase-free water containing 10% FBS or mouse serum, but relatively resistant to human serum ( Supplementary Fig. 6 ). In contrast, cM362-140 was quite stable under all these conditions. Thus, synthetic cM362-140 consisting of the cM362-capped RNA strand and antisense RNA strand was found to be more resistant to serum nucleases than cM362-139(IVT) consisting of three nucleotide strands. cM362-140 activates TLR3 but not cytoplasmic RNA sensors cM362-140 efficiently induced TLR3-dependent IFN-β promoter activation similar to cM362-139(IVT), when it was used to stimulate HEK293 cells expressing human TLR3 by simple addition or endosomal delivery ( Fig. 2a , left and centre panels). Activation of cytoplasmic RNA/DNA sensors by cM362-140 was hardly observed in HEK293 cells similar to cM362-139(IVT) ( Fig. 2a , right panel). To address the potential of cM362-140 for cytokine induction, splenic DCs from wild-type, Tlr3 −/− or Mavs −/− mice were stimulated with poly(I:C), cM362-139(IVT), control synthetic dsRNA140 or cM362-140, either alone or complexed with N-(1-(2,3-Dioleoyloxy)propyl)-N, N, N-trimethylammonium methyl-sulfate) (DOTAP) to deliver them to endosomes, or complexed with Lipofectamine to deliver them to cytoplasm. Extracellular addition of cM362-139(IVT) and cM362-140 to splenic DCs induced a subtle increase in TNF-α, IL-6 and IFN-β production compared with poly(I:C) treatment, whereas synthetic dsRNA140 (with no GpC) did not induce any cytokine over the detection limits ( Fig. 2b , left panels). Endosomal delivery of cM362-139(IVT) or cM362-140 with DOTAP also induced minimal levels of TNF-α, IL-6 and IFN-β dependent upon TLR3 ( Fig. 2b , centre panels). When the compounds were transfected into cytoplasm with Lipofectamine, MAVS-dependent cytokine production was barely observed with cM362-140, whereas only low levels of IL-6 and IFN-β were induced with cM362-139 in TLR3 KO DC ( Fig. 2b , right panel). This MAVS activity may reflect the exposure of a few 5′-triphosphated species of cM362-139(IVT) due to minor RNA degradation. These results indicate that cM362-140 targets endosomal TLR3 and activate the TICAM-1 pathway in both human and mouse cells. 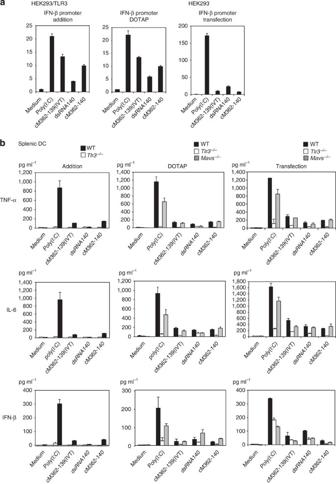Figure 2: TLR3-activating ability of cM362-140 in human and mouse cells. (a) TLR3-dependent IFN-β promoter activation by cM362-140. HEK293 cells were transiently transfected with IFN-β reporter and phRL-TK together with (left and middle panels) or without the expression plasmid for hTLR3 (right panel). Twenty-four hours after transfection, culture medium was removed and 10 μg ml−1poly(I:C), cM362-139(IVT), dsRNA140 or cM362-140 in fresh medium (left panel), or the same compounds complexed with DOTAP liposomal reagent (middle panel), or with Lipofectamine 2000 (right panel) were added to cells. Luciferase activity was measured 6 h (left and middle panel) or 24 h (right panel) after stimulation, and expressed as fold induction relative to the activity of non-stimulated cells. Representative data from three independent experiments, each performed in triplicate, are shown (mean ±s.d.). (b) Splenic CD11c+DCs (1.0 × 106per ml) isolated fromTlr3−/−,Mavs−/−or WT mice were stimulated with 10 μg ml−1untreated (left panels), DOTAP liposomal reagent-conjugated (middle panels) or Lipofectamine 2000-conjugated (right panel) nucleic acids as indicated. Twenty-four hours after stimulation, IFN-β in the culture supernatants was quantified using ELISA. TNF-α and IL-6 levels were measured using CBA. Representative data from three to five independent experiments are shown (mean±s.d.). Figure 2: TLR3-activating ability of cM362-140 in human and mouse cells. ( a ) TLR3-dependent IFN-β promoter activation by cM362-140. HEK293 cells were transiently transfected with IFN-β reporter and phRL-TK together with (left and middle panels) or without the expression plasmid for hTLR3 (right panel). Twenty-four hours after transfection, culture medium was removed and 10 μg ml −1 poly(I:C), cM362-139(IVT), dsRNA140 or cM362-140 in fresh medium (left panel), or the same compounds complexed with DOTAP liposomal reagent (middle panel), or with Lipofectamine 2000 (right panel) were added to cells. Luciferase activity was measured 6 h (left and middle panel) or 24 h (right panel) after stimulation, and expressed as fold induction relative to the activity of non-stimulated cells. Representative data from three independent experiments, each performed in triplicate, are shown (mean ±s.d.). ( b ) Splenic CD11c + DCs (1.0 × 10 6 per ml) isolated from Tlr3 −/− , Mavs −/− or WT mice were stimulated with 10 μg ml −1 untreated (left panels), DOTAP liposomal reagent-conjugated (middle panels) or Lipofectamine 2000-conjugated (right panel) nucleic acids as indicated. Twenty-four hours after stimulation, IFN-β in the culture supernatants was quantified using ELISA. TNF-α and IL-6 levels were measured using CBA. Representative data from three to five independent experiments are shown (mean±s.d.). Full size image In vivo cytokine induction by cM362-140 Injection of poly(I:C) into mouse peritoneal cavity strongly induced proinflammatory cytokine production in a TLR3-independent manner and high level of TNF-α and IL-6 were detected in sera at 3 h after injection ( Fig. 3a ). In contrast, both cM362-140 and cM362-139(IVT) hardly induced cytokine production and serum TNF-α, IL-6 and IL-10 levels were very low, which is mediated by TLR3 ( Fig. 3a ). Unlike poly(I:C), cM362-140 or -139(IVT) induced undetectable levels of IFN-β in wild-type mouse sera ( Supplementary Fig. 7 ). 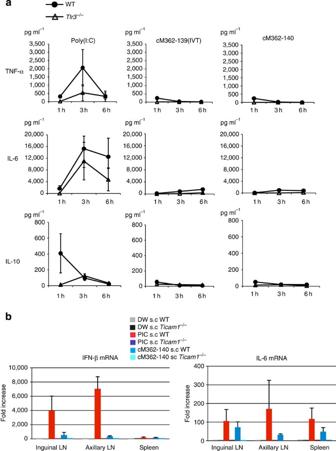Figure 3: cM362-139(IVT) and cM362-140 do not induce inflammatory cytokines. (a) Wild-type orTlr3−/−female mice (9 week) were injected i.p. with 50 μg poly(I:C), cM362-139(IVT) or cM362-140 in RNase-free water. At timed intervals, blood was collected from the tail vein and TNF-α, IL-6 and IL-10 levels in each sample were measured using a CBA. Data are shown as the mean±s.e.;n=3 mice per group. (b) Wild-type orTicam−/−female mice were injected s.c. with distilled water (DW), poly(I:C) or cM362-140 in RNase-free water. After 6 h, spleen, inguinal and axillary LNs were harvested andIFN-β andIL-6mRNA expressions were quantified by qPCR. Data are expressed as the fold induction relative to the expression in DW-injected mice and shown as the mean±s.e.;n=3 mice per group. Figure 3: cM362-139(IVT) and cM362-140 do not induce inflammatory cytokines. ( a ) Wild-type or Tlr3 −/− female mice (9 week) were injected i.p. with 50 μg poly(I:C), cM362-139(IVT) or cM362-140 in RNase-free water. At timed intervals, blood was collected from the tail vein and TNF-α, IL-6 and IL-10 levels in each sample were measured using a CBA. Data are shown as the mean±s.e. ; n =3 mice per group. ( b ) Wild-type or Ticam −/− female mice were injected s.c. with distilled water (DW), poly(I:C) or cM362-140 in RNase-free water. After 6 h, spleen, inguinal and axillary LNs were harvested and IFN -β and IL-6 mRNA expressions were quantified by qPCR. Data are expressed as the fold induction relative to the expression in DW-injected mice and shown as the mean±s.e. ; n =3 mice per group. Full size image A subcutaneous (s.c.) injection of cM362-140 induced the mRNAs of IFN-β and IL-6, but not TNF-α, in the inguinal and axillary lymph nodes (LNs) and spleen; the expression level was lower than that induced by poly(I:C) ( Fig. 3b ). These results suggest that TLR3-specific activation with cM362-140 results in low levels of cytokine production in vivo either by intraperitoneal (i.p.) or s.c. administration. EG7 tumour regression by CTL induced by cM362-139/140 The next question was whether cM362-139(IVT) causes tumour growth retardation as observed with poly(I:C). EG7 cells (a lymphoma cell line containing ovalbumin, OVA) were inoculated into the back of wild-type (WT) C57BL/6 mice, and the indicated materials were injected s.c. around the EG7 tumour that developed ( Fig. 4 ). Tumour growth was mildly retarded by treatment with poly(I:C) or cM362-139(IVT) alone ( Fig. 4a ). Combination therapy of OVA and poly(I:C) or cM362-139(IVT) resulted in complete remission of EG7 tumour >12 days after the treatment ( Fig. 4a ). The results infer that the combination of RNA adjuvant+tumour Ag exerts antitumour immune effect in spite of the low induction of proinflammatory cytokines. 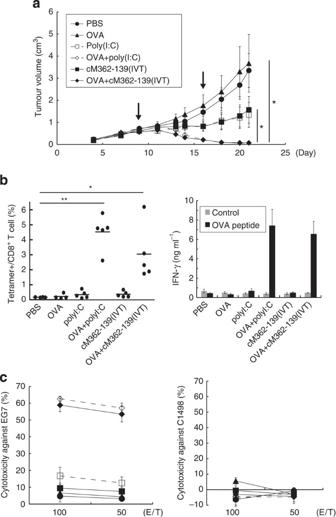Figure 4: cM362-139(IVT) induces CTL-mediated tumour regression. (a) Antitumour effect of cM362-139(IVT). WT mice were challenged with EG7 cells, and 7 and 14 days later they were s.c. injected with control PBS ([cirf ]), OVA (▴), polyI:C (□) and OVA+polyI:C (⋄) or cM362-139(IVT) (▪) or OVA+cM362-139 (♦). Tumour size was evaluated in each group. All error bars used in this figure show ±s.e.m. Data are representative of two independent experiments. Each group consisted of five mice. *P<0.05 (ANOVA with Bonferroni’s test). (b) OVA-specific CTL induction by cM362-139(IVT). Left panel: spleen cells were harvested at day 21 (7 days after 2nd therapy) and the proportion of tetramer-positive cells/CD8+T cells was evaluated. *P<0.05, **P<0.01. Right panel: spleen cells were harvested at day 21 as for the left panel. The cells were stimulated with OVA peptide for 3 days and the level of IFN-γ in the culture supernatant was measured. (c) Ag-specific cytotoxicity induced by cM362-139(IVT). Splenocytes collected from tumour-bearing mice at day 21 were cultured in the presence of immorbilized EG7 for 5 days. Then, the cytotoxicity against EG7 (left panel) or C1498 (control, right panel) was measured by51Cr release assay. Figure 4: cM362-139(IVT) induces CTL-mediated tumour regression. ( a ) Antitumour effect of cM362-139(IVT). WT mice were challenged with EG7 cells, and 7 and 14 days later they were s.c. injected with control PBS ([cirf ]), OVA ( ▴ ), polyI:C (□) and OVA+polyI:C ( ⋄ ) or cM362-139(IVT) (▪) or OVA+cM362-139 (♦). Tumour size was evaluated in each group. All error bars used in this figure show ±s.e.m. Data are representative of two independent experiments. Each group consisted of five mice. * P <0.05 (ANOVA with Bonferroni’s test). ( b ) OVA-specific CTL induction by cM362-139(IVT). Left panel: spleen cells were harvested at day 21 (7 days after 2nd therapy) and the proportion of tetramer-positive cells/CD8 + T cells was evaluated. * P <0.05, ** P <0.01. Right panel: spleen cells were harvested at day 21 as for the left panel. The cells were stimulated with OVA peptide for 3 days and the level of IFN-γ in the culture supernatant was measured. ( c ) Ag-specific cytotoxicity induced by cM362-139(IVT). Splenocytes collected from tumour-bearing mice at day 21 were cultured in the presence of immorbilized EG7 for 5 days. Then, the cytotoxicity against EG7 (left panel) or C1498 (control, right panel) was measured by 51 Cr release assay. Full size image We next tested whether s.c. injection of cM362-139(IVT) plus OVA induced CTL proliferation. The OVA tetramer assay and IFN-γ production were employed to evaluate OVA-specific CD8 + T-cell activation. Combination therapy of cM362-139(IVT) with OVA exhibited an increase in the frequency of Ag-specific CD8 + T cells comparable to poly(I:C) with OVA ( Fig. 4b ). Ag-specific CD8 + T cells clonally proliferated against EG7 as in vitro cytotoxicity was directed exclusively to EG7 in mice stimulated with cM362-139(IVT) with OVA ( Fig. 4c ) as well as poly(I:C) with OVA [9] . EG7 growth retardation by cM362-139(IVT) with OVA was largely abrogated in TLR3 KO mice ( Supplementary Fig. 8 ), suggesting that cM362-139(IVT) acts on host TLR3 in vivo . However, mild tumour growth retardation was still observed with cM362-139(IVT) with OVA in TLR3 KO mice ( Supplementary Fig. 8 ), implying minor involvement of EG7 cell TLR3 or other host RNA sensors, such as RLR [26] and DEAD-box helicases [27] , in in vivo tumour regression. Yet, tumor cell's TLR3 signaling and chemokine induction might affect tumor remission (refs 28 , 29 , 30 ). We finally tested whether chemically synthesized cM362-140 harbours the ability to retard EG7 growth in the same model. The synthetic cM362-140 showed ~80% activity for IFN-β reporter activation compared with cM362-139(IVT) and a single treatment with cM362-140 caused barely any regression of EG7 tumours in this model ( Fig. 5a ). Nevertheless, combination therapy with OVA+cM362-140 still induced tumour growth retardation ( Fig. 5a ). OVA-specific CD8 + T cells proliferated and activated in the mice stimulated with OVA+cM362-140, as assessed by tetramer assay ( Fig. 5b ) and IFN-γ production ( Fig. 5c ). We confirmed that the induction of OVA-specific CD8 + T-cell activation by cM362-140+OVA largely depends on TLR3/TICAM-1 using KO mice ( Supplementary Fig. 9 ). Although polyI:C induces RIP1/3-mediated necroptosis via TICAM-1 in some tumour lines, cM362-140 was not the case in EG7 tumour ( Supplementary Fig. 10 ). Hence, TLR3 has an important role in inducing cM362-140-mediated immune response and tumour growth retardation in the s.c. setting we employed in this study. 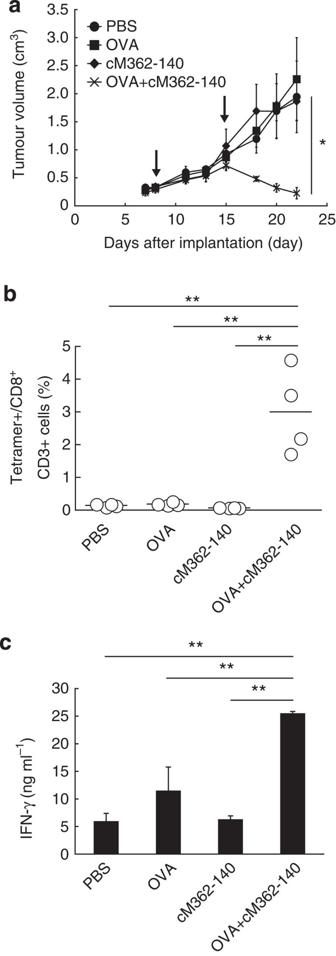Figure 5: cM362-140 induces EG7 tumour growth retardation. (a) Antitumour effect of cM362-140. As inFig. 4, tumour-bearing mice were s.c. injected with PBS, OVA, cM362-140 and OVA+cM362-140 at timed intervals (days 8 and 15). Tumour size was evaluated in each group. (b) OVA-specific CTL induction by cM362-140. The proportion of tetramer-positive cells/CD8+T cells in spleen was evaluated at day 22 (7 days after 2nd therapy). (c) Ag-specific IFN-γ production induced by cM362-140. Splenocytes were harvested at day 22 and incubated with OVA peptides for 3 days. The level of IFN-γ in the supernatant was measured by ELISA. *P<0.05, **P<0.01 (ANOVA with Bonferroni’s test). Figure 5: cM362-140 induces EG7 tumour growth retardation. ( a ) Antitumour effect of cM362-140. As in Fig. 4 , tumour-bearing mice were s.c. injected with PBS, OVA, cM362-140 and OVA+cM362-140 at timed intervals (days 8 and 15). Tumour size was evaluated in each group. ( b ) OVA-specific CTL induction by cM362-140. The proportion of tetramer-positive cells/CD8 + T cells in spleen was evaluated at day 22 (7 days after 2nd therapy). ( c ) Ag-specific IFN-γ production induced by cM362-140. Splenocytes were harvested at day 22 and incubated with OVA peptides for 3 days. The level of IFN-γ in the supernatant was measured by ELISA. * P <0.05, ** P <0.01 (ANOVA with Bonferroni’s test). Full size image Antigen-specific CD8 + T-cell priming by cM362-139/140 The Ag-specific CD8 + T-cell priming ability of cM362-139/140 in tumour-free settings was next examined using spleen and inguinal LN cells. Wild-type mice were injected s.c. with OVA with or without RNA adjuvants twice per week. Since OVA-specific CD8 + T cells most proliferated in spleen or inguinal LN 4 days after the last injection of OVA+poly(I:C) ( Fig. 6a ), spleen and LN cells were harvested from mice 4 days after the last adjuvant injection. cM362-139/140 significantly induced OVA-specific CD8 + T-cell proliferation in the inguinal LN and spleen compared with poly(I:C) ( Fig. 6b ). OVA-specific IFN-γ production in spleen cells was also efficiently induced by cM362-139(IVT) and cM362-140 ( Fig. 6c ). The TICAM-1 pathway was mainly involved in Ag-specific CD8 + T-cell activation induced by cM362-140 ( Fig. 6d ). 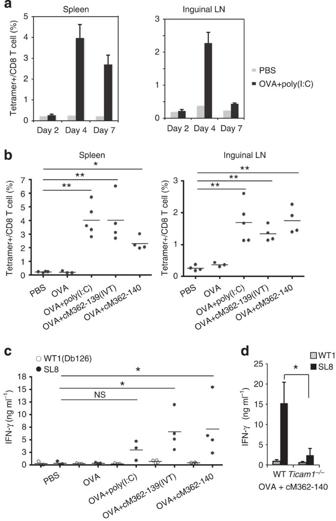Figure 6: cM362-139/140-induced antigen-specific CD8 T-cell activation in tumour-free settings. (a) Time-course experiments of poly(I:C)-induced antigen-specific CD8 T-cell activation in spleen and inguinal LN. WT mice were injected s.c. with 100 μl PBS or 50 μg poly(I:C)+100 ng OVA twice per week. Spleen and inguinal LN cells were harvested at 2, 4 or 7 days after the last adjuvant injection and an increase of OVA-specific CD8 T-cell proliferation was evaluated with tetramer assay. (b,c) WT mice were injected s.c. with PBS, OVA, OVA+50 μg poly(I:C), OVA+50 μg cM362-139(IVT) or OVA+70 μg cM362-140 twice per week. Spleen and inguinal LN cells were harvested 4 days after the last adjuvant injection and an increase of OVA-specific CD8 T-cell proliferation (b) and IFN-γ production (c) were then evaluated. (b) Proportion of tetramer-positive cells/CD8 T cells in spleen and inguinal LN. (c) Spleen cells were stimulated with OVA (SL8) or WT1 (Db126) peptide for 3 days and the level of IFN-γ in the culture supernatant was measured using a CBA. NS, no significant (>0.05), *P<0.05, **P<0.01, compared with PBS control (ANOVA with Dunnett’s test). (d) cM362-140+OVA induced Ag-specific CTL activation via the TICAM-1 pathway. Wild-type orTicam1−/−mice were injected s.c. with PBS, OVA or OVA+cM362-140 as described above. Spleen cells were harvested 4 days after the last adjuvant injection and OVA-specific IFN-γ productions were assessed. PBS or OVA injection did not induce IFN-γ production from spleen cells. The data from OVA+cM362-140 injection are shown. *P<0.05 (Student’st-test). Figure 6: cM362-139/140-induced antigen-specific CD8 T-cell activation in tumour-free settings. ( a ) Time-course experiments of poly(I:C)-induced antigen-specific CD8 T-cell activation in spleen and inguinal LN. WT mice were injected s.c. with 100 μl PBS or 50 μg poly(I:C)+100 ng OVA twice per week. Spleen and inguinal LN cells were harvested at 2, 4 or 7 days after the last adjuvant injection and an increase of OVA-specific CD8 T-cell proliferation was evaluated with tetramer assay. ( b , c ) WT mice were injected s.c. with PBS, OVA, OVA+50 μg poly(I:C), OVA+50 μg cM362-139(IVT) or OVA+70 μg cM362-140 twice per week. Spleen and inguinal LN cells were harvested 4 days after the last adjuvant injection and an increase of OVA-specific CD8 T-cell proliferation ( b ) and IFN-γ production ( c ) were then evaluated. ( b ) Proportion of tetramer-positive cells/CD8 T cells in spleen and inguinal LN. ( c ) Spleen cells were stimulated with OVA (SL8) or WT1 (Db126) peptide for 3 days and the level of IFN-γ in the culture supernatant was measured using a CBA. NS, no significant (>0.05), * P <0.05, ** P <0.01, compared with PBS control (ANOVA with Dunnett’s test). ( d ) cM362-140+OVA induced Ag-specific CTL activation via the TICAM-1 pathway. Wild-type or Ticam1 −/− mice were injected s.c. with PBS, OVA or OVA+cM362-140 as described above. Spleen cells were harvested 4 days after the last adjuvant injection and OVA-specific IFN-γ productions were assessed. PBS or OVA injection did not induce IFN-γ production from spleen cells. The data from OVA+cM362-140 injection are shown. * P <0.05 (Student’s t -test). Full size image NK cell-mediated B16 tumour regression by cM362-139/140 Using a C57BL/6-B16 syngeneic NK-sensitive tumour-implant model [9] , we evaluated NK-dependent antitumour activity of cM362-139(IVT) injected s.c. around the pre-formed tumour ( Fig. 7a ). Suppression of tumour growth, determined as reported previously [9] , was observed in the group that received cM362-139(IVT) compared with the water-treated group. The retardation of B16 tumour growth appeared to depend on TLR3 and TICAM-1 ( Fig. 7a,b ). NK1.1 + cells were involved in this tumour growth retardation ( Fig. 7c ), consistent with the NK-sensitive properties of B16 cells. No direct tumour cytolysis by macrophages [31] was associated with B16 growth retardation in the cM362-139(IVT) therapy. Splenocytes from the cM362-139(IVT)-treated group exerted higher cytotoxicity than those from the control group in vitro ( Fig. 7d ). 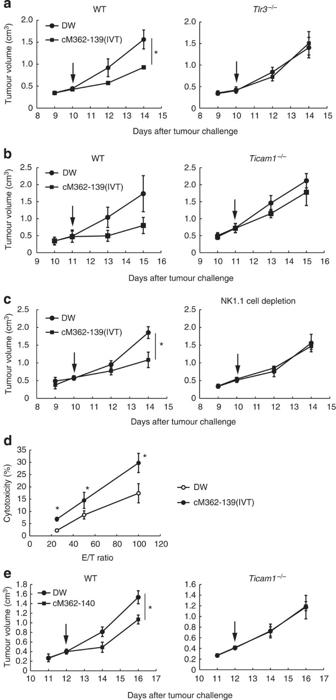Figure 7: Therapeutic effects of sODN-dsRNA in B16 tumour-implant model. (a,b) B16 tumour growth in mice after cM362-139(IVT) treatment. B16 melanoma cells were s.c. implanted into B6 WT mice (aandb),Tlr3−/−mice (a), orTicam1−/−mice (b). cM362-139(IVT) or distilled water was injected s.c. around the tumour on the day indicated by arrow and then tumour volume was measured. Data are shown as tumour average volume±s.e.;n=3 mice per group. *P<0.05. (c) Effect of NK cell depletion on cM362-139(IVT) treatment. Tumour-bearing mice were injected with anti-NK1.1 antibody to deplete NK cells. After 24 h, cM362-139(IVT) or distilled water was injected into the mice as described ina. (d) Cytotoxic activity of DX5+NK cells isolated from cM362-139(IVT)-treated mice. DX5+cells were isolated from B16 tumour-bearing mice treated with cM362-139(IVT) or distilled water for 18 h. Cytotoxic activity of DX5+cells against B16 target cells was measured by51Cr release assay. (e) B16 tumour growth in mice after cM362-140 treatment. Tumour-bearing mice were treated with cM362-140 as described ina. Figure 7: Therapeutic effects of sODN-dsRNA in B16 tumour-implant model. ( a , b ) B16 tumour growth in mice after cM362-139(IVT) treatment. B16 melanoma cells were s.c. implanted into B6 WT mice ( a and b ), Tlr3 −/− mice ( a ), or Ticam1 −/− mice ( b ). cM362-139(IVT) or distilled water was injected s.c. around the tumour on the day indicated by arrow and then tumour volume was measured. Data are shown as tumour average volume±s.e. ; n =3 mice per group. * P <0.05. ( c ) Effect of NK cell depletion on cM362-139(IVT) treatment. Tumour-bearing mice were injected with anti-NK1.1 antibody to deplete NK cells. After 24 h, cM362-139(IVT) or distilled water was injected into the mice as described in a . ( d ) Cytotoxic activity of DX5 + NK cells isolated from cM362-139(IVT)-treated mice. DX5 + cells were isolated from B16 tumour-bearing mice treated with cM362-139(IVT) or distilled water for 18 h. Cytotoxic activity of DX5 + cells against B16 target cells was measured by 51 Cr release assay. ( e ) B16 tumour growth in mice after cM362-140 treatment. Tumour-bearing mice were treated with cM362-140 as described in a . Full size image The chemically synthesized TLR3 ligand cM362-140 expressed a similar tumour-suppressing activity against B16 implant melanoma in the same model ( Fig. 7e ). This cM362-140-mediated NK-tumoricidal activity on B16 tumours was abrogated in Ticam1 −/− mice ( Fig. 7e ). Thus, cM362-140 suppresses NK-sensitive tumours in vivo via TLR3 by acting as an NK-inducing adjuvant. Cancer immunotherapy relies on suitable adjuvants. Many TAA peptides have been synthesized, but the lack of an appropriate adjuvant to induce an immune response against the peptides has hampered progress in peptide vaccine therapy. Although many candidates, most of which were retrospectively recognized as TLR agonists, have been tested in humans [1] , [6] , they have not yet been clinically approved because of their undesired effects. In this study, we designed many nucleotide adjuvants and tested their functional properties. Our approach is timely since most dsRNA receptors have been identified in the mouse and human [1] , [2] , [3] , [4] , and their structures and properties have been known for a decade [32] , [33] , [34] . Based on our current understanding of the dsRNA response, poly(I:C) activates both TICAM-1 (ref. 35 ) and MAVS pathways [36] resulting in systemic cytokinemia in mice [21] , [37] . Viral replication intermediates, double-stranded RNA and 5′-triphosphate RNA cause activation of the RLR pathway and robust cytokine production [38] , [39] . Here we chemically synthesized and tested a synthetic compound, cM362-140, an sODN-dsRNA that entered the endosomes and activated the TLR3/TICAM-1 pathway in vivo . Specifically, cM362-140 activated TLR3 in myeloid cells, including DCs in draining LNs, and induced activation of NK cells and proliferation of CTL. There was no systemically significant production of cytokines, including IFNs, after treatment with cM362-140. Our study establishes the proof-of-concept that modified or complexed RNA can regulate the immune response through TLR3 (refs 37 , 40 ), and that cM362-140 performs this function in vivo . In this study, a systemic increase in the cytokine levels was not required for the induction of an antitumour immune response. Instead, a basal cytokine level effectively primed DCs to activate tumoricidal NK cells and CTL response. Subcutaneous or i.p. injection of cM362-140 barely activated the RLR pathway, whereas poly(I:C) activated this pathway to induce systemic cytokinemia. cM362-140 activated TICAM-1 for DC maturation, but barely induced chemokine production or necroptosis in tumour cells ( Supplementary Fig. 10 ), which were reported as a direct action of poly(I:C) [29] , [30] . Therefore, cM362-140 eliminates major inflammatory responses caused by poly(I:C). The 5′-sODN sequence of cM362-140 targeted the dsRNA to the endosome and evaded recognition by RIG-I/MDA5. A 140-bp stretch of dsRNA was required for TLR3 multimerization and TICAM-1 activation, but unsatisfactory for endosome targeting [40] , [41] . The 5′-sODN sequence of cM362 does not contain a CpG motif, which stimulates cytokine production via TLR9 in plasmacytoid DC. To prevent Dicer-mediated RNA interference, RNA sequences specific to human mRNAs were not employed. In addition, the antisense 5′-end of cM362-140 was OH, neither phosphorylated nor capped, unlike viral or host RNA products. Although cM362-140 was an artificial compound to circumvent host innate sensors, its constituents are native and modifiable to maximize antitumour response. Although the nucleic acid-sensing system differs somewhat between mouse and human [2] , [4] : generally, human BDCA3 + DCs express a high level of TLR3 but no TLR9 (ref. 20 ), whereas mouse CD8α + DCs express TLR3 and TLR9 (refs 2 , 18 , 41 ), extrapolating results from the mouse and applying them to the human will be crucial for establishing human immunotherapy in the future. Type I IFNs have remarkable antiviral and antitumour properties, but sometimes elicit severe side effects during treatment in patients. For example, s.c. injection of poly(I:C) induces inflammation, erythema and fever [42] . In clinical trials, cancer patients cannot tolerate high doses of poly(I:C), even if administered via s.c. injection [11] , [40] , [41] , [42] . Poly(I:C) consists of polyI and polyC chains of variable lengths that differ in function from one batch to the next, and, for unknown reasons, exogenous poly(I:C) activates cytoplasmic RNA sensors [36] . By contrast, cM362-140 is uniform. It binds TLR3 and fails to activate cytoplasmic RNA sensors, indicating that immune modulation by RNA occurs only in the draining LNs and tumour microenvironment [45] . Thus, cM362-140 enables us with a ‘defined’ immunotherapy to patients without systemic cytokine response or inflammation. Several compounds that activate the TICAM-1 pathway are clinically available. Monophosphoryl lipid A is a TLR4 adjuvant that activates the TICAM-2/TICAM-1 cascade via TLR4/MD-2 (ref. 46 ). However, monophosphoryl lipid A still retains the TLR4-mediated MyD88 activation, which conceptually different from sODN-dsRNA that activates a single cascade of PRR. Although poly(A:U) mildly activates the TLR3 pathway and induces type I IFN in humans [47] , it has far less adjuvancy than poly(I:C) [6] , [28] , [48] . In a short-term clinical trial, poly(I:C 12 U), also known as ampligen, has been shown to be less toxic than other immunotherapies [49] , [50] . Unfortunately, data on its uniformity and TLR3-specificity as an adjuvant are scant. Poly(I:C)LC, another antitumour adjuvant, has shown clinical promise, but it causes cytokine toxicity, thereby precluding its further development [5] , [6] , [42] , [43] , [44] , [51] . Type I IFN induction and the output of IFNAR activation appear to be predominant in low-dose poly(I:C) administration in human volunteers [42] . In another clinical study, a low dose (1.4 mg per body) of poly(I:C)LC in combination with NY-Eso-1, which contains TAA epitopes, has been shown to mount a tumour-specific T-cell response [11] . Although low doses of poly(I:C)LC induce type I IFN, it only insufficiently stimulates T-cell proliferation in vivo [11] . cM362-140 is advantageous over poly(I:C)LC in that a high dose can be used to specifically activate TICAM-1, but not MAVS in vivo . This is the first report of the successful chemical creation of a long, sequence-defined and bioactive TLR3-specific ligand. The targeting of programmed cell death-1 and cytotoxic T-lymphocyte-associated protein-4 with monoclonal antibodies in patients with progressive-staged cancer may provide another immunotherapy breakthrough [52] . Except for an alum adjuvant that can induce a Th2 response [2] , [53] , there is no suitable adjuvant-TAA combination for immunotherapy. Immune enhancing by adjuvant would be required since tumour cells can undergo mutations and survive to circumvent immune attack. A main problem is that current adjuvant candidates are all inflammatory, facilitating formation of tumour-supporting microenvironment, that accelerates genome instability, tumour growth and progression [45] . Here, sODN-dsRNA is a non-inflammatory adjuvant sustaining DC-mediated NK/CTL activation, its combining with TAAs will bring a therapeutic benefit to a number of patients with intractable tumours. Cell culture, reagents and plasmid HEK293 cells were maintained in Dulbecco's Modified Eagle's medium (Invitrogen) supplemented with 10% heat-inactivated FCS (Invitrogen) and antibiotics. HeLa cells were kindly provided by Dr T. Fujita (Kyoto University) and maintained in Eagle’s minimal essential medium (Nissui,) supplemented with 1% L -glutamine and 5% FCS. B16D8 melanoma cells were cultured at 37 °C under 5% CO 2 in RPMI containing 10% FCS, penicillin and streptomycin. EG7 and C1498 cells were purchased from ATCC and cultured in RPMI-1640 supplemented with 10% FCS, 55 μM 2-mercaptoethanol (2-ME) and 1 mM sodium pyruvate, and RPMI-1640 supplemented with 10% FCS and 25 ng ml −1 2-ME, respectively. Poly(I:C) was purchased from Amersham Biosciences. Endotoxin-free ovalbumin was purchased from Hyglos. OVA 257-264 peptide (SL8), control WT1 peptide (Db126) and OVA (H2K b -SL8) tetramer were from MBL. Human serum type AB was from Lonza. ODNs were synthesized by GeneDesign. Following antibodies were used in this study: Alexa Fluor-568-conjugated secondary antibody (Invitrogen), FITC-CD8α (53-6.7) and APC-CD3ε (145-2C11) (BioLegend), and PerCP/Cy5.5-7AAD (BD Biosciences). The human TLR3 expression plasmid was constructed in our laboratory [33] . Preparation of in vitro transcribed sODN-dsRNAs The leader-trailer sequence of a MV laboratory-adapted strain of Edmonston was used as the dsRNA template [25] . DNA fragments covering this region of the MV genome and the T7 promoter sequence were amplified using PCR with specific primers and the plasmid pCR-T7 MV as a template. Sense and antisense MV RNAs from the PCR products were in vitro transcribed using an AmpliScribe T7 transcription kit (Epicentre Technologies) according to the manufacturer’s protocol. The transcribed products were purified by 8% PAGE containing 7 M urea. After visualization by ultraviolet illumination, the appropriate bands were excised and eluted with 0.3 M sodium acetate. The eluted RNAs were ethanol precipitated and resuspended in RNase-free water. For large-scale preparation of RNAs, electro-elutions were performed using D-Tube Dialyzer Maxi (Novagen) and eluted RNAs were dialyzed, concentrated and precipitated with ethanol. The concentration of RNA was determined by measuring the absorbance at 260 nm in a spectrophotometer. To generate sODN-dsRNA, sODN+linker DNA, sense and antisense RNA were mixed and annealed. sODNs, MV RNA sequences in sODN-dsRNA and PCR primers used in this study are described in Supplementary Tables 1–3 . Preparation of cM362-140 The chemically synthesized long RNAs as an alternative to in vitro transcribed RNAs were completed by a ligation reaction mediated by splint DNA [54] with slight modification. The outline of chemical synthesis was described below. To prepare the sense strand of cM362-140, the ligation reactions were performed in two steps. First, S2 RNA (40 nmol), S3 RNA (40 nmol) and specific splint DNA (40–48 nmol) were mixed, heated at 90 °C for 5 min and slowly cooled to 4 °C ( Supplementary Table 4A,B ). Following hybridization, T4 DNA ligase (Takara) was added and incubated at room temperature for 16–22 h. The ligation reaction mixtures comprised 15.4 μM annealed complex, 66 mM Tris-HCl (pH 7.6), 6.6 mM MgCl 2 , 10 mM DTT, 0.1 mM ATP and ~31 U μl −1 T4 DNA ligase. As the second ligation, S1 cM362-RNA (40 nmol) and the specific splint DNA (40–48 nmol) for the second ligation site were added into the first ligation reaction mixture, hybridized and T4 DNA ligase was added. The mixture was incubated at room temperature for 16–22 h. The derived full-length 165 mer sense strand was isolated by 8% PAGE containing 7 M urea and electro-elution. The subsequent procedure was the same as described in the section describing purification of in vitro transcribed RNAs. Overall yield was 8–10%. To prepare the antisense RNA of cM362-140, three fragment RNAs, AS1, AS2 and AS3 (33 nmol each) and the related splint DNAs (33 nmol each) were mixed, hybridized and then T4 DNA ligase was added. The mixture was incubated at room temperature for 16–22 h. The following procedure was the same as described above. Overall yield was 15–22%. To generate cM362-140, sense- and antisense-RNAs were annealed. Analysis with microchip electrophoresis To analyse the cM362-139 complex, we used a microchip electrophoresis instrument (model SV1210; Hitachi Electronics Engineering Co. Ltd.). The standard procedure for electrophoresis using 2-mercaptoethanol (ME) has been previously described [55] , [56] . sODN or RNAs were adjusted to 0.2 μM with water. The sODN/RNA1/RNA2 complex (designated cM362-139) and dsRNA (RNA1+RNA2) were prepared by mixing DNA or RNAs and hybridizing in water (final concentration 0.4 μM). The sample solution (10 μl) was applied to the sample well of the microchip device and the programme was run at 600 V for 120 s (injection time), then at 1,100 V for 180 s (separation time) under 350 V of return voltage at 20 °C. During the electric separation, DNA or RNA peaks were detected by laser induced fluorescence and analysed. Agarose gel electrophoresis cM362-139(IVT) and cM362-140 were incubated in PBS or in RNase-free water with or without serum, for 60 min at 37 °C or 42 °C. Aliquots containing 0.1–0.2 μg of incubated sODN-dsRNAs were then mixed with 10 × loading dye (Takara Bio Inc.) and loaded onto 3 or 4% agarose gel (Nusieve 3:1 Agarose, Lonza) containing ethidium bromide. After electric separation, nucleic complexes were visualized using ultraviolet transilluminator (FAS-III, Toyobo). Reporter gene assay HEK293 cells (8 × 10 5 cells per well) were cultured in six-well plates and transfected with the TLR3 expression vector or empty vector (400 ng per well) together with the reporter plasmid (400 ng per well) and an internal control vector, phRL-TK (Promega; 20 ng per well) using Lipofectamine 2000 (Invitrogen). The p-125 luc reporter containing the human IFN-β promoter region (−125 to +19) was provided by Dr T. Taniguchi (University of Tokyo). Twenty-four hours after transfection, cells were collected and resusupended in medium with or without FCS. Then, cells were seeded into 96-well plates and stimulated with the indicated RNAs for 6 h. The Firefly and Renilla luciferase activities were determined using a dual-luciferase reporter assay kit (Promega). The Firefly luciferase activity was normalized to the Renilla luciferase activity and was expressed as the fold induction relative to the activity in unstimulated vector-transfected cells. All assays were performed in triplicate. Cytokine assay Splenic CD11c + DCs from wild-type, Tlr3 −/− or Mavs −/− mice were prepared as described previously [9] , [31] . Cells were suspended in RPMI-1640 (Invitrogen) supplemented with 10% heat-inactivated FCS and antibiotics and stimulated with the indicated RNAs. Twenty-four hours after stimulation, culture supernatants were collected and analysed for cytokine levels by ELISA or Cytometric Bead Array (CBA). ELISA kits for mouse IFN-α and IFN-β were purchased from PBL Biomedical Laboratories. CBA flex sets for mouse IL-6 and TNF-α were purchased from BD Bioscience. Experiments were performed according to the manufacturer’s instructions and samples were analysed using the Facs Aria (BD Bioscience). Confocal microscopy HeLa cells (1.0 × 10 5 cells per well) were cultured on microcover glasses (Matsunami Glass Ind., Ltd) in a 12-well plate. Three hours after seeding, cells were transfected with GFP-fused Rab5a or Lamp1 using BacMam systems (Cell Light Early Endosomes-GFP BacMam 2.0 or Cell Light Lysosomes-GFP BacMam 2.0, Life technologies) or left untreated. Sixteen hours after transfection, cells were incubated with 15 μg ml −1 Cy3-labelled cM362, cM362-dsRNAs or dsRNAs for 30 min at 4 °C. Cells were washed twice and further incubated at 37 °C. And then, cells were fixed with 4% paraformaldehyde at the time points indicated. The coverslips were mounted onto slide glass with Prolong Gold with DAPI for nuclei staining. Cells were visualized at a × 63 magnification using a Zeiss LSM520 META microscope (Carl Zeiss Microscopy GmbH). Quantitative PCR (qPCR) Total RNA was extracted using the Trizol reagent (Qiagen) and reverse-transcribed using a high-capacity cDNA Reverse Transcripition kit (Applied Biosystems) and random primers according to the manufacturer’s instructions. QPCR was performed using specific primers for mouse GAPDH, IFN -β, IL-6 and TNF -α ( Supplementary Table 5 ) and the Step One Real-time PCR system (Applied Biosystems). Mice Ticam1 −/− and Mavs −/− mice were made in our laboratory and backcrossed more than eight times to adapt C57BL/6 background [9] , [10] . Inbred C57BL/6 WT mice were purchased from CLEA Japan. Tlr3 −/− mice were kindly provided by Dr S. Akira (Osaka University). Mice were maintained under specific pathogen-free conditions in the animal facility of the Hokkaido University Graduate School of Medicine. Female mice 6–12 weeks of age were used in all experiments, all of which were performed according to the guidelines issued by the Hokkaido University Animal Care and Use Committee. In vivo mouse cytokine assay Wild-type and Tlr3 −/− mice (9 weeks) were injected i.p. with 50 μl (50 μg) poly(I:C), cM362-139 (IVT) or cM362-140, and blood was collected from the tail vein at timed intervals. Cytokine levels in sera were measured using a CBA. In some cases, wild-type and Ticam1 −/− mice were s.c. injected with 75 μl (75 μg) poly(I:C) or cM362-140. After 6 h, mice were killed and draining inguinal LN, axillary LN and spleen were harvested [10] . IFN -β, IL -6 or TNF -α mRNA expression in these lymphoid organs was measured by qPCR. Tumour challenge and sODN-dsRNA treatment Mice 6–10 weeks of age were used in all experiments. Mice were shaved at the back and injected s.c. with 200 μl of 6 × 10 5 B16D8 cells in PBS (−). Tumour volumes were measured at regular intervals using a caliper [9] . Tumour volume was calculated using the following formula: tumour volume (cm 3 )=(long diameter) × (short diameter) 2 × 0.4. 75 μl (75 μg) sODN-dsRNAs or distilled water with no detectable LPS was mixed with in vivo -JetPEI (Polyplus), a polymer-based transfection reagent, according to the manual and then injected s.c. around the tumour. Treatment was started when the average tumour volume of 0.4–0.6 cm 3 was reached. To deplete NK cells, we injected titrated anti-NK1.1 ascites (PK136) i.p. in tumour-bearing mice the day before sODN-dsRNA treatment. Depletion of NK1.1 + cells was verified by flow cytometory. In the case of EG7 cell challenge, mice were injected s.c. with 200 μl of 2 × 10 6 syngenic EG7 cells in PBS (−). When the average tumour volumes reached ~0.6 cm 3 , 50 μl of 100 μg endotoxin-free ovalbumin in PBS (−) with or without 50 μl of 50 μg poly(I:C) or sODN-dsRNA was injected s.c. around the tumour. PBS (−) (100 μl) was used as a control. Treatments were performed twice per week. CTL activity in tumour-bearing mice after adjuvant therapy Female mice 6–10 weeks of age were used for this study. Splenocytes were harvested from tumour-bearing mice at 7 days after the last adjuvant treatment. In the case of tumour-free settings, spleen and inguinal LN cells were harvested from wild-type or Ticam1 −/− mice 4 days after the last adjuvant injection. The cells were stained with FITC-CD8α (1:200), PerCP/Cy5.5-7AAD (1:200), APC-CD3ε (1:200) and PE-OVA-tetramer (1:50) to detect Ag-specific CD8 + T cells. To evaluate cytokine production, splenocytes (2 × 10 6 per 200 μl per well) were cultured for 3 days in the presence of 100 nM OVA peptide (SL8: SIINFEKL) or control WT1 peptide (Db126: RMFPNAPYL) and IFN-γ production was analysed with CBA or ELISA. To assess the cytotoxic activity of CTLs, splenocytes (1 × 10 6 per ml) were co-cultured with mitomycin C-treated EG7 cells (5 × 10 5 per ml) in the presence of 10 U ml −1 IL-2 for 5 days. Then, the cells were incubated with 51 Cr-labelled EG7 or C1498 cells for 4 h and determined cytotoxic activity [10] . The cytotoxicity was calculated by this formula: Cytotoxicity (%)=[(experimental release−spontaneous release)/(total release—spontaneous release)] × 100. Cytotoxic activity assay of NK cells Mice bearing B16 tumour were injected s.c. with cM362-139(IVT) mixed with in vivo -JetPEI. After 18 h, mice were killed and DX5 + NK cells were isolated from spleen using DX5-positive selection microbeads (Miltenyi) according to the manual [9] . B16 cells were labelled with 51 Cr for 1 h and then washed three times with medium. DX5 + cells and 51 Cr-labelled B16 cells were co-cultured at the indicated ratio [31] . After 4 h, supernatants were harvested and 51 Cr release was measured in each sample. Specific lysis was calculated by the following formula: cytotoxicity (%)=[(experimental release−spontaneous release)/(total release−spontaneous release)] × 100. Statistical analysis The significance of differences between groups was determined by the Student’s t -test. In tumour-implant or -free mouse experiments, one-way analysis of variance with Bonferroni’s multiple-comparison test or Dunnett’s test was performed to analyse statistical significance. How to cite this article : Matsumoto, M. et al . Defined TLR3-specific adjuvant that induces NK and CTL activation without significant cytokine production in vivo . Nat. Commun. 6:6280 doi: 10.1038/ncomms7280 (2015).